Ligand substitutions between ruthenium–cymene compounds can control protein versus DNA targeting and anticancer activity Ruthenium compounds have become promising alternatives to platinum drugs by displaying specific activities against different cancers and favourable toxicity and clearance properties. Nonetheless, their molecular targeting and mechanism of action are poorly understood. Here we study two prototypical ruthenium-arene agents—the cytotoxic antiprimary tumour compound [(η 6 - p -cymene)Ru(ethylene-diamine)Cl]PF 6 and the relatively non-cytotoxic antimetastasis compound [(η 6 - p -cymene)Ru(1,3,5-triaza-7-phosphaadamantane)Cl 2 ]—and discover that the former targets the DNA of chromatin, while the latter preferentially forms adducts on the histone proteins. Using a novel ‘atom-to-cell’ approach, we establish the basis for the surprisingly site-selective adduct formation behaviour and distinct cellular impact of these two chemically similar anticancer agents, which suggests that the cytotoxic effects arise largely from DNA lesions, whereas the protein adducts may be linked to the other therapeutic activities. Our study shows promise for developing new ruthenium drugs, via ligand-based modulation of DNA versus protein binding and thus cytotoxic potential, to target distinguishing epigenetic features of cancer cells. Metal-based compounds, such as cisplatin, carboplatin and oxaliplatin, are among the most widely used chemotherapeutic agents [1] , [2] . The therapeutic effect of these classic platinum drugs is mediated by formation of DNA lesions, which appear to interfere mainly with transcription resulting in apoptosis. However, there is limited effectiveness due to severe toxicity and intrinsic or acquired resistance issues [3] . Indeed, the small size and square planar geometry of the platinum species yields only modest site discrimination in reaction with the double helix, with adducts forming preferentially at the most solvent accessible guanine nucleotides [4] . The limitations associated with traditional platinum agents and improved knowledge of tumour biology has prompted renewed interest in the development of alternative metal-based anticancer compounds [5] . Ruthenium agents have been showing great promise from their selective activity against specific cancer cells types in combination with low toxicity, and two compounds are presently in clinical trials [6] . Moreover, the octahedral bonding of both Ru(II) and Ru(III) species affords an extensive repertoire of three-dimensional architectures, giving the potential for a high degree of site selectivity and implementation of favourable pharmacological attributes. Nonetheless, relatively little is known about the molecular targeting characteristics and mechanism of action of ruthenium agents. Although it is traditionally assumed that DNA is the pharmacological target, recent evidence suggests that, at least for certain compounds, proteins are likely involved in the therapeutic effect [7] , [8] , [9] , [10] . However, chemical attributes that could distinguish the DNA versus protein targeting are not known. A caveat of many in vitro studies on the molecular targeting of reactive metal species is that most can form adducts on isolated guanine bases or oligonucleotides in solution, whereas in the cell site selectivity is governed by the outcome of competition between many different kinds of molecules. Moreover, the packaging of the genome by histone proteins into nucleosomes can alter the adduct formation potential of different DNA sites [11] . We earlier found that the ruthenium antimetastasis agent [(η 6 - p -cymene)Ru(1,3,5-triaza-7-phosphaadamantane)Cl 2 ] [12] , [13] (RAPTA-C; Fig. 1 ) accumulates on cellular chromatin, potentially forming adducts at specific histone sites on the nucleosome core [8] . This suggested that RAPTA-C may primarily target proteins, but it was unclear whether adduct accumulation on chromatin in the cell was primarily associated with the histone or the DNA component. Intriguingly, while RAPTA-C is inactive against primary tumours, it is able to inhibit both the spreading and growth of metastases in mice and also has anti-angiogenic properties [13] , [14] . Indeed with its low cell-killing potential, whereby growth inhibition assays of RAPTA-C have yielded IC 50 values of >300 μM for both normal and cancer cell lines [13] , RAPTA-C would not be considered cytotoxic in standard compound screening assays [15] . 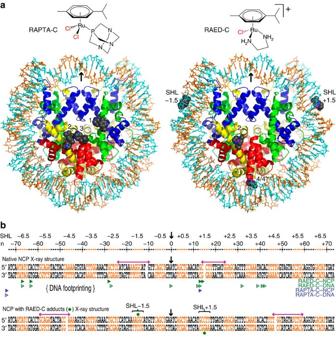Figure 1: Ruthenium compound site selectivity. (a) Chemical structures and nucleosomal adducts of RAPTA-C and RAED-C. X-ray structures of adducted NCP are shown looking down the DNA superhelical axis, with the nucleosome pseudo-twofold axis running vertically (arrow). Histone proteins are shown in blue (H3), green (H4), yellow (H2A) and red (H2B), and the two 145-nucleotide DNA strands are cyan and orange. RAPTA-C and RAED-C adducts appear with space-filling representation (sites 1–4, histone associated; sites SHL ±1.5, DNA associated). (b) DNA structure and sequence preference of adduct formation. Orange and black lettering for the DNA sequence designates regions where the minor as opposed to the major groove, respectively, face inward towards the histone octamer in the NCP. Severe kinks at locations of DNA stretching around SHL ±2 or ±5 (magenta arrows) result in a shift in the histone-DNA register, depicted as a gap in the sequence. The footprinting analysis of naked and nucleosomal DNA, shown inFig. 3, is summarized with exonuclease stop sites depicted as arrowheads, adjacent to the terminal 3′ nucleotide, pointing towards the ruthenium adduct. Filled and open symbols correspond to very strong and moderate termination points, respectively. Figure 1: Ruthenium compound site selectivity. ( a ) Chemical structures and nucleosomal adducts of RAPTA-C and RAED-C. X-ray structures of adducted NCP are shown looking down the DNA superhelical axis, with the nucleosome pseudo-twofold axis running vertically (arrow). Histone proteins are shown in blue (H3), green (H4), yellow (H2A) and red (H2B), and the two 145-nucleotide DNA strands are cyan and orange. RAPTA-C and RAED-C adducts appear with space-filling representation (sites 1–4, histone associated; sites SHL ±1.5, DNA associated). ( b ) DNA structure and sequence preference of adduct formation. Orange and black lettering for the DNA sequence designates regions where the minor as opposed to the major groove, respectively, face inward towards the histone octamer in the NCP. Severe kinks at locations of DNA stretching around SHL ±2 or ±5 (magenta arrows) result in a shift in the histone-DNA register, depicted as a gap in the sequence. The footprinting analysis of naked and nucleosomal DNA, shown in Fig. 3 , is summarized with exonuclease stop sites depicted as arrowheads, adjacent to the terminal 3′ nucleotide, pointing towards the ruthenium adduct. Filled and open symbols correspond to very strong and moderate termination points, respectively. Full size image In the present study, we established that the chromatin-bound adducts in cancer cells treated with RAPTA-C are primarily associated with the protein component, not the DNA. Since related ruthenium compounds are believed to preferentially target DNA, we wanted to determine whether this is the case, and if so, to establish the basis for such differential molecular discrimination. We found that [(η 6 - p -cymene)Ru(ethylenediamine)Cl]PF 6 (refs 16 , 17 ) (RAED-C; Fig. 1a ) does preferentially target the DNA component of chromatin in cells. In contrast to RAPTA-C, RAED-C displays high cytotoxicity and antiprimary tumour activity analogous to that of cisplatin, and we employed structural, computational and analytical methodologies to understand the basis for the surprisingly different activities of these two structurally related ruthenium agents. Protein versus DNA targeting We used inductively coupled plasma mass spectrometry (ICP-MS) to characterize the localization of RAED-C and RAPTA-C in cancer cells ( Table 1 ). 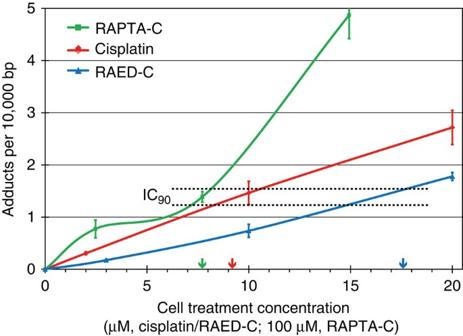Figure 2: DNA–metal adduct levels in treated A2780 cancer cells. Arrows indicate IC90values for RAPTA-C (green; 772 μM), cisplatin (red; 9.2 μM) and RAED-C (blue; 17.6 μM). The interpolated agent concentration values for cisplatin (9.5±1.0 μM) and RAED-C (16.3±1.6 μM) that would yield the same adduct levels corresponding to the IC90for RAPTA-C are within error equal to the respective IC90values of the two agents (dashed lines provide approximate frame; mean±s.d.,n=3). Subsequent to incubation of cells with the two agents at their respective IC 50 values ( Table 2 ), ~33 × 10 6 and ~250 × 10 6 molecules of RAED-C and RAPTA-C, respectively, are taken up per cell. Of the total intracellular ruthenium content, 8% for RAED-C compared with 4% for RAPTA-C is associated with the chromatin. Of these chromatin-bound adducts, the majority is associated with the DNA component for RAED-C (~77%), whereas for RAPTA-C, the majority (~61%) is associated with the protein component (from ratios of DNA:chromatin adducts in Table 1 ). Table 1 Ruthenium compound-binding behaviour. Full size table Table 2 Cell growth inhibition values ( μ M). Full size table To shed further light on the proclivity of both agents to amass adducts within the nuclei of cancer cells, we employed size exclusion chromatography-ICP-MS to characterize reactivity towards the nucleosome core—the basic element of histone-packaged DNA. RAED-C and RAPTA-C both react rapidly with nucleosome core particle (NCP) in solution to yield stable adducts, with respective association constants of 6.7 × 10 5 and 2.3 × 10 5 M −1 ( Table 1 ). However, compared with RAPTA-C, for which ~85% of the adducts are associated with the histone proteins, RAED-C reacts threefold faster with ~71% of adducts associated with the DNA. 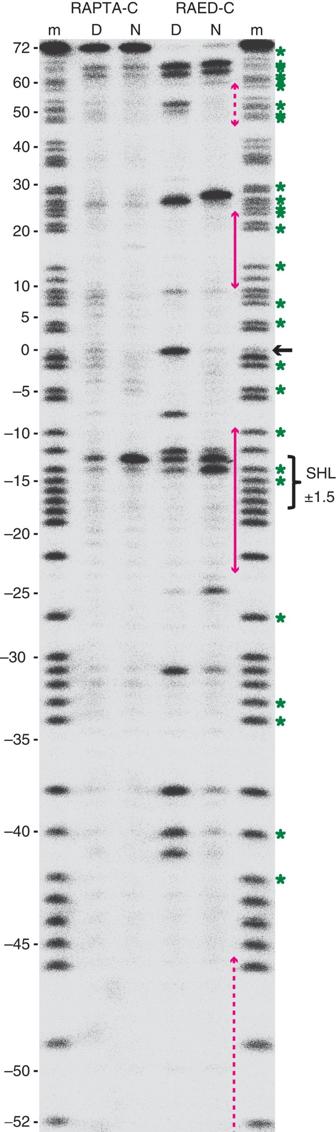Figure 3: Exonuclease digest analysis reveals DNA–ruthenium adduct formation profiles. DNA samples, consisting of either NCP (N) or the corresponding naked DNA (D) treated with RAPTA-C or RAED-C, are shown with purine sequencing standards (m). Numbers represent nucleotide position relative to the nucleosome centre (black arrow), green asterisks designate the locations of guanine nucleotides and magenta arrows indicate regions of DNA stretching in the native (solid) and RAED-C adducted (dashed) NCP structures. Effectively, the same site selectivity difference between the two compounds is apparent over the 10-fold range of agent:NCP molar stoichiometry tested ( Table 3 ), indicative of a fundamental site preference distinction. In addition, DNA adduct levels measured following cellular uptake continue to increase in a linear or exponential manner at concentrations well above the IC 50 values of RAED-C and RAPTA-C ( Fig. 2 ), indicating an absence of site saturation for DNA binding. Table 3 Adduct formation in the nucleosome core. Full size table Figure 2: DNA–metal adduct levels in treated A2780 cancer cells. Arrows indicate IC 90 values for RAPTA-C (green; 772 μM), cisplatin (red; 9.2 μM) and RAED-C (blue; 17.6 μM). The interpolated agent concentration values for cisplatin (9.5±1.0 μM) and RAED-C (16.3±1.6 μM) that would yield the same adduct levels corresponding to the IC 90 for RAPTA-C are within error equal to the respective IC 90 values of the two agents (dashed lines provide approximate frame; mean±s.d., n =3). Full size image The protein versus DNA preference based on isolated nucleosome core reactivity is in excellent agreement with the cellular localization results. In fact, the slightly higher fraction of both RAED-C and RAPTA-C adducts associated with the DNA for the cellular chromatin analysis suggests a greater reactivity of the protein-free, or linker, DNA that connects adjacent nucleosome core regions in the genome (see below)—a phenomenon that has been found for platinum drugs and other types of small molecules [11] , [18] . DNA sequence and histone packaging modulate site selectivity Previous studies have shown that RAED-C forms adducts at guanine bases of oligonucleotide DNA [19] , [20] and that RAPTA-C also binds to DNA [12] . However, since DNA structure, flexibility, sequence context and histone packaging can influence platinum drug site selection [4] , [21] as well as adduct formation by non-metal-based compounds that also attack guanine N7 groups [22] , we wanted to determine whether these factors also influence ruthenium agent reaction. We had previously established a DNA footprinting assay based on exonuclease digestion to analyse platinum compound site selection and cross-link generation for both the naked and nucleosomal states of the double helix [4] , [21] . The enzyme digests a single strand of double helical DNA in the 3′–5′ direction, and we found here that, like for platinum lesions, digestion is also arrested on encountering ruthenium compound adducts ( Figs 1b and 3 ). Figure 3: Exonuclease digest analysis reveals DNA–ruthenium adduct formation profiles. DNA samples, consisting of either NCP (N) or the corresponding naked DNA (D) treated with RAPTA-C or RAED-C, are shown with purine sequencing standards (m). Numbers represent nucleotide position relative to the nucleosome centre (black arrow), green asterisks designate the locations of guanine nucleotides and magenta arrows indicate regions of DNA stretching in the native (solid) and RAED-C adducted (dashed) NCP structures. Full size image The nuclease digestion DNA footprint for naked DNA and NCP treated with RAED-C reveals selective adduct formation at guanine nucleotides, but with an apparent favouring of GG dinucleotide sites suggesting a contribution of electrostatic attraction in governing reactivity, as observed for simple metal hydrates. Strikingly, however, the site selectivity of the naked compared with the nucleosomal state is dramatically different, with most of the reactive sites on naked DNA being protected by histone packaging. The only sites of substantial adduct formation are within the last double helical turn at the termini and at locations 1.5 and 2.5 double helical turns from the nucleosome centre (SuperHelix Location (SHL) ±1.5 and SHL ±2.5). Moreover, although the two terminal digest arrest locations are identical between the naked and nucleosomal states, this is not the case for the SHL ±1.5 and ±2.5 regions, which display elevated reactivity in the nucleosome and single nucleotide differences in adduct location between the two states. This indicates that histone packaging can generate hotspots for ruthenium agent adduct formation as well as shift inherent reactivity from one guanine to an adjacent base. For RAPTA-C, it is difficult to obtain a strong DNA footprint because of its low intrinsic reactivity for the double helix ( Figs 1b and 3 ). In fact, a substantial portion of the material contains RAPTA-C adducts at the DNA termini, yielding an undigested 145 bp fragment. However, as there are effectively no DNA termini in vivo , this is an artefact that suggests a steric challenge behind RAPTA-C adduct formation on the double helix. Nonetheless, albeit weak, the RAPTA-C footprint shows similar guanine site selectivity in comparison with that of RAED-C. Notably, there is a single strong site of RAPTA-C adduct formation aside from the termini, which occurs for the nucleosomal state at SHL ±1.5—analogous to the strongest site of adduct formation observed for RAED-C. Nucleosome structure governs adduct formation In a recent X-ray crystallographic study of RAPTA-C binding to the NCP, we identified three sites of specific adduct formation that entail bivalent coordination to glutamate, histidine and lysine side chains of the histone proteins [8] ( Fig. 1a ). 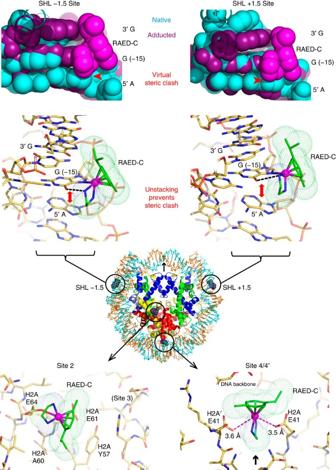Figure 4: Crystal structure of RAED-C adducts on the DNA and histones in the nucleosome core. At top, the two symmetry-related DNA adduct sites (magenta) are shown in comparison with the respective native NCP structure (cyan; models were superimposed with respect to the guanine bases to which RAED-C coordinates and are shown with space-filling representation). Hydrogen bonding between the ethylenediamine ligands and adducted guanine bases is indicated with dashed lines (middle). Site 4/4′ of the histone adducts (bottom right) entails binding along the pseudo-twofold axis of the nucleosome (black arrow), coinciding with a crystallographic mixture of monofunctional binding to glutamate 41 of either copy of H2A. RAED-C treatment of NCP crystals also results in adduct formation at two different histone sites, one of which (site 2) is common to both agents, but in contrast to RAPTA-C, adducts on the DNA are also observed ( Figs 1 and 4 ; Table 4 ; Supplementary Fig. 1 ). The DNA adducts occur at two pseudo-symmetry-related locations, SHL ±1.5, and entail monofunctional coordination to the 5′-guanine N7 atom of an AGG element ( Fig. 4 ). The cymene and ethylenediamine groups of RAED-C form extensive van der Waals contacts with the bases to the 5′ and 3′ sides of the coordinating guanine as well as with the sugar-phosphate backbone. In addition, a hydrogen bond occurs between the O6 atom of the coordinating guanine and the proximal amine group of the ethylenediamine ligand. Figure 4: Crystal structure of RAED-C adducts on the DNA and histones in the nucleosome core. At top, the two symmetry-related DNA adduct sites (magenta) are shown in comparison with the respective native NCP structure (cyan; models were superimposed with respect to the guanine bases to which RAED-C coordinates and are shown with space-filling representation). Hydrogen bonding between the ethylenediamine ligands and adducted guanine bases is indicated with dashed lines (middle). Site 4/4′ of the histone adducts (bottom right) entails binding along the pseudo-twofold axis of the nucleosome (black arrow), coinciding with a crystallographic mixture of monofunctional binding to glutamate 41 of either copy of H2A. Full size image Table 4 Data collection and refinement statistics for NCP treated with RAED-C. Full size table The carrier ligands of RAED-C in the guanine adducts appear to form favourable interactions with the double helix, but the conformation of the DNA around both adduct sites is in fact dramatically different compared with the native NCP structure ( Figs 1b and 4 ). In untreated NCP crystals, the double helix displays stretch distortions over SHL ±1.5 (ref. 23 ), which renders the DNA susceptible to attack at these locations. DNA stretching, characterized by elongation and overtwisting of the double helix, is an intrinsic property of the nucleosome that is influenced by DNA sequence and exogenous factors, such as metal binding [4] , [24] , [25] . The extreme kinking and other deformations associated with stretching over SHL ±1.5 yield exceptional steric access to the 5′-guanine N7 groups of the AGG elements [4] . Although these native-state conformations favour RAED-C attack, they are incompatible with the adducted state since a steric clash would occur between the ethylenediamine group and the adenine base to the 5′-side if there were not a conformational rearrangement. The solution adopted is for the DNA stretching to relocate to the alternative location around the SHL ±5 regions, which allows the double helix at SHL ±1.5 to assume a conformation compatible with the RAED-C adducts. Interestingly, although the structures of the AGG elements are very different between the two pseudo-symmetry-related SHL −1.5 and SHL +1.5 halves in the native state, they become nearly identical in the adducted state. This indicates an intrinsically favoured adduct configuration, which notably entails a pronounced asymmetric base–base unstacking distortion relative to the 5′-adenine that allows steric accommodation of the ethylenediamine group. Steric factors dictate the distinct reactivity Although the histone protein site discrimination of RAPTA-C and RAED-C is similar, with both agents preferentially forming adducts on glutamate, their very different DNA versus protein adduct formation potential suggests that the ethylenediamine and phosphaadamantane ligands are decisive in governing molecular targeting. To understand the basis for this distinction, we employed hybrid quantum mechanical/molecular mechanical (QM/MM) calculations. This approach allowed us to study the adduct formation process even for the nucleosome core system in its entirety (~200 kDa+solvent) by treating all residues, with the exception of those directly involved in adduct formation, with the relatively computationally inexpensive MM potential. We started by performing QM calculations of the structures and energetics associated with RAED-C and RAPTA-C reacting at isolated amino acids and nucleotides corresponding to the histone glutamate (site 2) and SHL ±1.5 DNA guanine sites common to both agents ( Supplementary Fig. 2 ) as indicated by the crystal structure and DNA footprinting analyses. However, this simplified system cannot explain the observed differences in the adduct formation potential between RAED-C and RAPTA-C, but suggests that the two compounds are electronically very similar and that distinctions in site preference involve structural/dynamic features of the macromolecular context. We subsequently performed QM/MM calculations on the reaction of RAED-C and RAPTA-C with the explicitly solvated NCP ( Fig. 5 ; Supplementary Fig. 3 and Supplementary Movies 1–4 ). Whereas the two compounds present a similar free energy barrier of about 20 kcal mol −1 for their reaction with the histone site, that associated with adduct formation on the DNA site is roughly twofold higher for RAPTA-C compared with RAED-C ( Supplementary Fig. 3 ). The activation barrier for RAED-C reaction with DNA is slightly lower than for the histone site, but in either case proceeds via an associative mechanism resulting in departure of the water ligand ( Fig. 5 ). 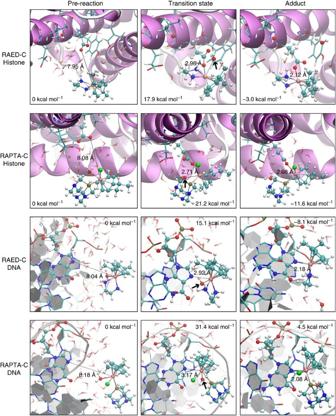Figure 5: Structure and energetics for the reaction of RAED-C and RAPTA-C at histone glutamate and DNA guanine sites in the nucleosome core. The structures were extracted from QM/MM simulations performed on explicitly solvated NCP in the presence of the ruthenium agents. The relative free energies (kcal mol−1) were calculated from constrained QM/MM simulations of the NCP by integrating the force acting along the reaction coordinate, which corresponds to the developing coordinate-covalent bond between ruthenium and either a glutamate carboxylate oxygen or guanine N7 atom (distances shown). H2O leaving groups are indicated with arrows. Figure 5: Structure and energetics for the reaction of RAED-C and RAPTA-C at histone glutamate and DNA guanine sites in the nucleosome core. The structures were extracted from QM/MM simulations performed on explicitly solvated NCP in the presence of the ruthenium agents. The relative free energies (kcal mol −1 ) were calculated from constrained QM/MM simulations of the NCP by integrating the force acting along the reaction coordinate, which corresponds to the developing coordinate-covalent bond between ruthenium and either a glutamate carboxylate oxygen or guanine N7 atom (distances shown). H 2 O leaving groups are indicated with arrows. Full size image Adduct formation mechanisms analogous to those for RAED-C were found for the reaction of RAPTA-C with the histone glutamate as well as the DNA guanine sites ( Fig. 5 ). However, in contrast to the accessible histone sites on the surface of the nucleosome, steric constraints in the double helix pose an obstacle towards accommodating both the cymene and phosphaadamantane ligands for the RAPTA-C adduct, and the resulting high energy pseudo-pentacoordinated transition state is reflected in the less favourable orientation that must be adopted by the cymene ligand and increased length of the incipient Ru–N adduct bond relative to the RAED-C transition structure ( Fig. 5 ). As a consequence of the steric obstacles, the activation barrier for RAPTA-C binding to the DNA is increased considerably and the stability of the final adduct is diminished as well, giving rise to both a kinetically and thermodynamically unfavourable free energy profile. For the above calculations, we studied the reactions of the mono-aquated states for both RAED-C and RAPTA-C. However, RAPTA-C contains a second chloride leaving group and can thus potentially undergo an additional aquation event to produce the di-aquated state, but solution studies of RAPTA-C have shown that the mono-aquated form is the most abundant species [26] . Here we also find with QM simulations that the mono-aquated form of RAPTA-C is far more energetically favourable (by 17 kcal mol −1 ) than the di-aquated species ( Supplementary Fig. 4 ). Nonetheless, we carried out QM calculations of RAPTA-C adducts at both glutamate and guanine sites to compare the energetics between the mono- and di-aquated reactant species ( Supplementary Fig. 5 ). Although the adduct stability for both the protein and the DNA sites are increased by the corresponding substitution of H 2 O in place of Cl − with respect to the reaction of the di-aquated species, the stability of the protein adduct is still more favourable in either case. This further indicates that the steric bulk of the phosphaadamantane ligand is the primary factor that distinguishes the histone/DNA site selectivity behaviour between RAPTA-C and RAED-C. Distinct activities in cancer cells Given the differences in site selectivity between RAED-C and RAPTA-C, we conducted cellular impact experiments in comparison with cisplatin to shed light on how differences in molecular targeting and adduct characteristics may give rise to the pharmacological distinctions between these three compounds. We treated standard and cisplatin-resistant human ovarian cancer cell lines, A2780 and cisplatin-resistant A2780 (crA2780), respectively, with drug for 24 h and followed the effects on cellular death and on the cell cycle directly thereafter (day 1), in addition to the following two days ( Fig. 6 ). This allowed us to assess not only differences in how cells are affected by but also recover from treatment. 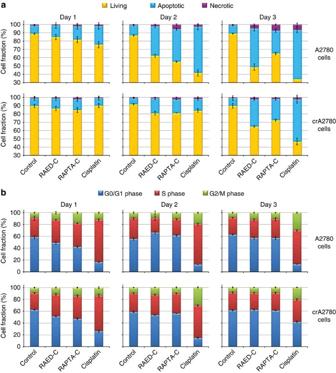Figure 6: Impact of ruthenium agents and cisplatin on cell viability and function. (a) Apoptosis/necrosis profiles derived from flow cytometric analysis of cultured cells. (b) Cell cycle profiles based on flow cytometric analysis of cultured cells. Day 1 measurements were made immediately after switching cells to agent-free media (subsequent to 24 h incubation with agent), and day 2 and day 3 measurement correspond to cells residing in agent-free media for an additional 1 or 2 days (mean±s.d.,n=3). Figure 6: Impact of ruthenium agents and cisplatin on cell viability and function. ( a ) Apoptosis/necrosis profiles derived from flow cytometric analysis of cultured cells. ( b ) Cell cycle profiles based on flow cytometric analysis of cultured cells. Day 1 measurements were made immediately after switching cells to agent-free media (subsequent to 24 h incubation with agent), and day 2 and day 3 measurement correspond to cells residing in agent-free media for an additional 1 or 2 days (mean±s.d., n =3). Full size image Considering the profound cytotoxicity distinction of RAPTA-C relative to RAED-C and cisplatin, we also quantified DNA adducts after 24-h exposure of A2780 cells to different concentrations of the three compounds ( Fig. 2 ). Notably, DNA–metal levels are closely linked to the respective cell growth inhibiting power of the different agents. In particular, the amount of DNA adducts measured for RAPTA-C, RAED-C and cisplatin are approximately equal at their respective IC 90 concentrations. This implies that the effect of all three agents on cell killing and growth inhibition arises primarily from the adducts formed on DNA, and the cell cycle and death analyses were also performed with the same degree and duration of treatment with compound. To understand the magnitude and significance of variations in the cell death and cell cycle profiles, we used a multivariate analysis method developed by Mahalanobis [27] . The Mahalanobis distances designate levels of dissimilarity between any two variable pairs, to which degrees of statistical confidence can be assigned. This analysis shows that the apoptosis and cell cycle profiles between the control and cisplatin-, RAED-C- and RAPTA-C-treated cells are highly distinct, with most of the functionally relevant parameter pairs having P values <0.0001 (from the Fisher distances, n =3; Supplementary Data 1 ). In addition, the cell impact profiles for the three compounds between the standard and resistant cell lines are distinct, while the behaviour of the two types of control cells is very similar ( Supplementary Data 1I,J ). This shows a differential impact of all three agents on A2780 compared with crA2780 cells. However, the relative differences, both in terms of apoptotic as well as cell cycle arrest profiles, are much more pronounced for cisplatin compared with either RAED-C or RAPTA-C. This is consistent with the virtual lack of cross-reactivity with cisplatin for the ruthenium compounds (see below). Relative to cisplatin, which has a blatant and long-lasting effect on cellular function, surviving cells recover more quickly after RAED-C or RAPTA-C treatment ( Fig. 6 ). Cisplatin-treated cells display a jump in extent of apoptosis well above that seen for the ruthenium agents 24 h (A2780 cells, day 2) or 48 h (crA2780 cells, day 3) after drug removal, and RAPTA-C even shows a decrease in apoptosis level by day 3, for A2780 cells ( Fig. 6a and Supplementary Data 1B,D ). Moreover, cell cycle profiles for RAED-C and RAPTA-C are more similar to control cells subsequent to drug removal by day 2 or day 3 ( Fig. 6b and Supplementary Data 1F,H ). Cisplatin is known to induce initial S-phase arrest as a DNA replication blockade is encountered, which is subsequently circumvented and followed later by increased G2/M phase arrest corresponding to transcriptional inhibition. In contrast, the ruthenium agents do not display this signature and instead elicit a degree of S-phase and G2/M-phase arrest that tends to diminish rapidly following drug removal ( Fig. 6b and Supplementary Data 1E–H ). Compared with the 14-fold cisplatin resistance level of the crA2780 relative to the A2780 cells, RAED-C and RAPTA-C display only a slight degree of cross-resistance, 1.5-fold and 2.1-fold, respectively (based on IC 50 values, Table 2 ). Some low level of cross-resistance seems also apparent in the fact that the cell cycle impact of RAED-C and RAPTA-C, like cisplatin, diminishes more rapidly following drug removal for the crA2780 compared with the A2780 cells ( Fig. 6b and Supplementary Data 1F,H ). On the other hand, whereas cisplatin relative to RAED-C and RAPTA-C induces more rapid apoptosis in A2780 cells, the impact potential is reversed in crA2780 cells, with RAED-C and RAPTA-C appearing to induce a faster apoptotic response ( Fig. 6a and Supplementary Data 1A–D ). Moreover, cisplatin has a diminished capacity to induce S-phase arrest relative to G2/M-phase arrest in the crA2780 compared with the A2780 cell lines, and this pattern is in fact the opposite of what is seen for RAED-C and RAPTA-C, which yield greater S-phase relative to G2/M-phase arrest in the resistant cell line ( Fig. 6b and Supplementary Data 1E,G,J ). In addition to the pronounced distinctions relative to cisplatin, differences in cellular impact between RAED-C and RAPTA-C are also apparent. In particular, RAPTA-C is more effective than RAED-C at inducing rapid G2/M-phase arrest ( Fig. 6b and Supplementary Data 1E–H ). One potential advantage of existing metal-based anticancer agents is that a given compound has the capacity to form adducts at many different therapeutic sites, including targets foundational to cell survival like DNA. This may permit superior efficacy by diminishing the likelihood of resistance gain. However, effective design of improved drugs will depend on determining where adducts are generated inside cells and which of the many adducts that form are therapeutic versus counterproductive or ineffective. This knowledge of site preference and mechanism of action would allow one to selectively target weak points of cancer cells, diminishing impact on healthy tissue. Since they display low toxicity and favourable clearance properties, in addition to non-cross-resistance attributes, ruthenium agents have become promising alternatives to platinum drugs [5] , [6] . Although RAED-C has been reported to display no cross-resistance relative to cisplatin towards cisplatin-resistant cancer cell lines [17] , we found here a slight level of cross-resistance for both RAED-C and RAPTA-C. However, magnitude of cross-resistance to different DNA-damaging agents has been shown to depend critically on the extent to which cells are resistant to cisplatin [28] . For instance, whereas (cr)A2780 cells that are only 7.3-fold resistant to cisplatin are not cross-resistant to adriamycin, those that are 14-fold resistant to cisplatin (an identical level of resistance as the crA2780 cells used in our study) display a 3.4-fold cross-resistance to this DNA intercalator. Moreover, other compounds, such as the nitrogen mustard alkylating agent melphalan, can display even greater levels of differential cross-resistance between the less and more cisplatin-resistant cell lines (2.1- versus 8.7-fold). In fact, the most chemotherapy-resistant cell lines may provide superior models for tumour biology, as these represent the most life-threatening cell types. Therefore, the mere approximately twofold level of cross-resistance found here for RAED-C and RAPTA-C with respect to highly cisplatin-resistant cells is striking considering that much greater degrees of cross-resistance are seen for unrelated (non-metal-based) DNA-damaging agents. This is encouraging since it suggests that the activity of ruthenium agents has little overlap with the mechanisms that can protect cancer cells from cisplatin and even other DNA-damaging compounds. Relative to RAPTA-C, which preferentially forms protein adducts in the cell, the activity of RAED-C is overall more similar to cisplatin, both in terms of DNA-targeting proclivity and apoptosis profile ( Fig. 6 and Supplementary Data 1A,C ). This supports the premise that RAED-C and cisplatin share high cytotoxicity and antiprimary tumour activity by virtue of their DNA lesion formation potential. However, the basal level of cross-resistance and the distinct cellular impact between cisplatin and RAED-C suggest that differences in DNA site preference and adduct structure are consequential. In this regard, RAED-C displays elevated DNA site selectivity over the classic platinum drugs, which form adducts at essentially any solvent-exposed guanine bases in the nucleosome core [4] . In contrast, RAED-C tends to form adducts only at the most distorted regions within the nucleosome core. Interestingly, in spite of this greater discrimination, an even larger fraction of RAED-C that is taken up by the cell ends up as DNA adducts, 6.4% ( Table 1 ), compared with 4.1% of cisplatin [10] . In addition, whereas the bifunctional adducts of cisplatin cause extreme kinking of the double helix, RAED-C produces monofunctional adducts that result in a much more subtle distortion of the DNA. These conformational differences in the double helix and distinctions in the steric bulk of the adducts apparently underlie the lower nucleotide excision repair efficiency observed for RAED-C relative to cisplatin adducts in vitro [20] and are also likely to yield differential effects on transcription factor binding and polymerase activity. Thus, there are substantial distinctions in DNA-targeting potential as well as localization and structure of the DNA adducts that form in the genome, which may account for differences in impact on cell cycle and mode of cell death between RAED-C and cisplatin by influencing adduct recognition and repair. One striking feature from the cellular studies is that both standard and cisplatin-resistant cancer cells recover substantially more quickly from RAPTA-C or RAED-C treatment compared with cisplatin exposure. This is especially intriguing considering that the cell treatment conditions yield roughly the same number of initial DNA adducts (at day 1) for all three compounds. Considering that the bonding strength of platinum is higher than that of ruthenium compounds due to greater covalent character of the adduct bonds would suggest that greater lability of the ruthenium adducts allows these lesions to clear more quickly subsequent to drug exposure. This may contribute to the favourable clearance and diminished toxicity properties of ruthenium agents and consequently suggests that optimizing, as opposed to maximizing, adduct stability may be a means for achieving the greatest differential impact between cancer and normal cells. In this sense, in conjunction with their elevated site discrimination potential, ruthenium compounds may offer a window of moderate-to-low cytotoxicity for cancer cell types or contexts where the high toxicity/potency of platinum drugs is not suited. Metastasis is arguably the most serious challenge for anticancer therapies, since it accounts for 90% of cancer deaths [29] . Unlike for eradicating tumour cells, an effective antimetastasis agent need not have cell-killing potential. In fact, a more readily achievable compromise may be met by looking for non-toxic agents that inhibit just the metastatic process itself, in particular since metastatic cells are especially resistant to apoptosis making them likely to be amongst the least affected by (nonspecific) cytotoxic compounds [30] . In this regard, the properties so far displayed by RAPTA-C are encouraging. In contrast to RAED-C, the low cytotoxic potential of RAPTA-C is consistent with the very high concentrations of the agent required to produce significant levels of DNA adducts. Changing the ethylenediamine ligand of [Ru-cymene-Cl] + to phosphaadamantane (+ Cl − ) switches the adduct formation profile from primarily targeting the DNA to the proteins associated with chromatin, and it is the sterically more demanding phosphaadamantane group that is responsible for inhibiting DNA adduct generation by increasing the reaction activation barrier and destabilizing the adducted product. This suggests new avenues to modulate DNA-targeting activity, and thus cytotoxic potential, through conservative alterations in carrier ligand structure. Nevertheless, in spite of the established distinctions in molecular targeting, it is possible that the mono-versus-bifunctional difference in coordination ability between RAED-C and RAPTA-C also contributes to their differential activity profiles. In this sense, RAPTA-C has the potential to form cross-links in and between proteins and nucleic acids, and whether such bonding is of functional significance remains to be determined. Although the mechanism behind the antimetastasis activity of RAPTA-C is not yet clear, it appears that protein targets are most probably involved. Since RAPTA-C has a particular proclivity to accumulate adducts at chromatin-associated proteins, it is interesting to speculate that histone lesions may contribute to the efficacy of this agent. The distinct profile of RAPTA-C for inducing rapid G2/M-phase arrest could be associated with such binding activity and suggests possibilities for novel combination anticancer therapies employing both histone- and DNA-targeting compounds. However, since almost 96% of the RAPTA-C adducts that form inside the cell are at non-chromatin sites, additional protein targets may well be relevant. The traditional definition of the cancerous state as arising from purely genetic abnormalities is now amended to entail epigenetic changes as critical elements in the oncogenic process [31] , [32] . Thus, cancer cells can be characterized by numerous, yet gene-specific, structural and chemical abnormalities in chromatin, which include distinctions in chromatin compaction status, nucleosome organization, DNA methylation, histone variant composition and post-translational modification of histones. In fact, recent work shows that subpopulations of drug-resistant cancer cells are even established via epigenetic modifications of chromatin [33] . The ability of RAPTA-C and RAED-C to recognize not just chemical but structural features of nucleosomes holds promise for targeting epigenetic weak points of cancer cells and suggests that these ruthenium agents and other compounds may achieve their therapeutic effects serendipitously through such activity. For instance, RAED-C adduct formation is dependent on double helix distortions in the nucleosome core and could thus be sensitive to differences in nucleosome positioning in the genome. Moreover, a remarkable feature of RAPTA-C is that it preferentially forms adducts at histone protein sites residing on the surface of the nucleosome core [8] . These include regions known to be important in chromatin compaction and protein factor association that are key transactions in gene regulation and cell division. As such, adduct formation at these histone regulatory sites could be sensitive to histone composition and compaction status of nucleosomes. Further characterization of the epigenetic vulnerabilities of cancer cells with improved understanding of metallocompound targeting and mode of action should yield superior drugs. Ruthenium compound synthesis RAPTA-C and RAED-C were synthesized as described previously [12] , [16] . In brief, for the synthesis of RAPTA-C, equimolar amounts of 1,3,5-triaza-7-phosphatricyclo[3.3.1.1]decane and [Ru(η 6 - p -cymene)Cl 2 ] 2 were refluxed in methanol, and the product was precipitated by addition of diethyl ether. RAED-C was prepared by stirring the methanol solution of [Ru(η 6 - p -cymene)Cl 2 ] 2 with an excess of ethylenediamine. Pure crystalline product was obtained by addition of NH 4 PF 6 and reducing the volume to 75–90%. The purity of the prepared products was confirmed through elemental analysis. Cellular uptake experiments Human A2780 ovarian carcinoma cells were obtained from the European Centre of Cell Cultures (Salisbury, UK) and maintained in culture as described by the provider. The cells were grown at 37 °C and 5% CO 2 in RPMI 1640 medium containing 10% FCS with 2 mM glutamine, 100 units ml −1 penicillin and 100 μg ml −1 streptomycin. The A2780 cells were seeded in six-well plates, grown to ~50% confluency and incubated with RAED-C or RAPTA-C at concentrations of 5 μM or 250 μM (corresponding to their IC 50 values; Table 2 ), respectively, for 24 h at 37 °C. At the end of the incubation period, the cells were washed three times with ice-cold PBS before being detached using an enzyme-free dissociation solution (Millipore, Switzerland). The cells were then centrifuged for 5 min at 700 g and 4 °C and washed twice with ice-cold PBS. Cell lysis was achieved using a freeze-thaw technique that was recently found to be suitable for cell uptake studies [34] . All samples were analysed for their protein content before ICP-MS determination using a bicinchoninic acid assay (Sigma-Aldrich, Switzerland). Chromatin isolation Chromatin isolation was achieved with a Pierce Chromatin Prep Module (26158; Thermo Scientific, Switzerland). Cells were grown in 75 cm 2 flasks to ~80% confluence before being incubated for 24 h at 37 °C with RAED-C or RAPTA-C at concentrations of 5 μM or 250 μM, respectively. At the end of the incubation period, cells were washed three times with ice-cold PBS to remove unbound drug, and the chromatin extract was prepared in accordance with the protocol supplied by the manufacturer. The determination was carried out as three independent experiments. DNA isolation Isolation of genomic DNA was carried out using a GenElute Mammalian Genomic DNA Miniprep Kit (G1N70; Sigma-Aldrich, USA). For the measurements in Table 1 , cells were grown in 25 cm 2 flasks to ~80% confluency before being incubated with RAED-C or RAPTA-C at concentrations of 5 μM or 250 μM, respectively, for 24 h at 37 °C. For the measurements in Fig. 2 , cells (obtained from the Health Protection Agency Culture Collections, Salisbury, UK) were grown in 60 mm plates to ~90% confluency before being incubated with 3/10/20 μM RAED-C, 247/772/1493 μM RAPTA-C or 2/10/20 μM cisplatin for 24 h at 37 °C. The amount of DNA was quantified by ultraviolet absorption measurements at 260 nm and subjected to ICP-MS analysis. Determination of binding constants X-ray crystallographic, DNA footprinting and analytical analysis of NCP and corresponding naked DNA were conducted using a 145-bp DNA fragment and nucleosome assembled with recombinant histones [23] . Samples containing 20 mM K-cacodylate (pH 6.0), 5 μM NCP and RAED-C:NCP ratios of 1:1, 2:1, 4:1 and 10:1 were incubated at room temperature for up to 48 h. Kinetic experiments of samples containing a 2:1 RAED-C:NCP ratio were carried out to determine the rate constant of the binding reaction (by monitoring the NCP–RAED-C adduct peak area) and the time required for an equilibrium to be established. The rate constant k was determined assuming pseudo-first-order kinetics and the binding constant K by using the equation r =( nKc )/(1+ Kc ) ( r , bound drug:NCP molar ratio; n , number of binding sites; c , concentration of unbound drug) [35] . The equation was solved for different RAED-C:NCP ratios by nonlinear regression analysis using Polymath 6.1. To assess the distribution of RAED-C adducts between the histone proteins and DNA of the nucleosome core, RAED-C-treated NCP was first dissociated with the addition of NaCl to a final concentration of 2.5 M before size exclusion chromatography (SEC) fractionation. ICP-MS measurements All determinations of metal content were conducted by monitoring the 102 Ru signal on an Elan DRC II ICP-MS instrument (Perkin Elmer, Switzerland) equipped with a Meinhard nebulizer and a cyclonic spray chamber or a 7700x Agilent ICP-MS instrument (Agilent Technologies, CA, USA) equipped with a MicroMist glass concentric nebulizer and a quartz Peltier-cooled spray chamber. For determination of the ruthenium or platinum content in the chromatin or DNA extracts, all samples were digested in concentrated ultrapure nitric acid (Sigma-Aldrich, Switzerland) for 3 h and the final volume adjusted with the addition of ultrapure water. Indium was added at a concentration of 0.5 p.p.b. as an internal standard. For SEC-ICP-MS measurements, a Perkin Elmer Series 200 HPLC-system was directly coupled to the Elan DRC II instrument. Twenty microlitres of sample was injected, and separations were achieved on a TSKGel SW guard column (Tosoh Biosciences, Germany) at a flow rate of 0.8 ml min −1 using 100 mM ammonium acetate running buffer. The ICP-MS instrument was tuned using a solution provided by the manufacturer containing 1 p.p.b. each of Mg, In, Ce, Ba, Pb and U. External standards were prepared gravimetrically in identical matrix to the samples (with regard to internal standard and nitric acid) with single element standards obtained from CPI International (Amsterdam, The Netherlands). The SEC columns were calibrated using a molecular weight calibration mixture with a range of 5–700 kDa (Sigma-Aldrich, Switzerland). DNA footprinting analysis Exonuclease III footprinting experiments for obtaining RAED-C and RAPTA-C adduct formation profiles, based on digest (3′–5′ direction) termination at DNA lesion sites, were conducted in a similar manner as described previously for platinum adduct mapping [4] , [21] . Five micromolar naked DNA or NCP in a buffer of 20 mM K-cacodylate (pH 6.0) was incubated at room temperature for 24 h with a 10-fold molar excess, for naked DNA, or a 20-fold molar excess, for NCP, of RAED-C or RAPTA-C. Samples were treated by heating at 55 °C with the addition of 4 M NaCl to a final concentration of 2 M, followed by phenol-chloroform extraction and ethanol precipitation of the DNA, which was then 5′-end-labelled ( 32 P) with polynucleotide kinase. Six hundred and seventy-five nanograms of DNA samples were subjected to digestion with 250 units of exonuclease III for 1 h, which is a 10-fold excess over that minimally required for full digestion of the untreated DNA. After ethanol precipitation, digested DNA samples were subsequently stripped of ruthenium adducts by treatment with 1 M thiourea for 16 h at 58 °C, followed again by ethanol precipitation of the DNA. Modified Maxam–Gilbert purine sequencing standards were prepared initially as described [36] , whereby DNA was 5′-end-labelled ( 32 P) with polynucleotide kinase, followed by treatment of 10 μl of the DNA (~100 μg ml −1 ) with 25 μl of 80% (v/v) formic acid. The reaction was halted after an incubation of 4–8 min by addition of 200 μl stop buffer (0.3 M Na-Acetate, 0.1 M EDTA, 25 μg ml −1 RNA), followed immediately by addition of 750 μl cold ethanol. After 10 min incubation on ice, the DNA was pelleted by centrifugation. The DNA pellet was then dissolved in 200 μl of 10% (v/v) piperidine, and the sample was incubated at 95 °C. The reaction was stopped after 45 min by ethanol precipitation of the DNA. Finally, DNA markers were subjected to 3′-dephosphorylation by treatment with 1 unit of polynucleotide kinase per 20 ng DNA for 16 h. The ethanol precipitated DNA marker pellet was resuspended by the addition of ~10 μl of loading dye and heating at 95 °C for 3 min. All DNA fragments were resolved by denaturing polyacrylamide gel electrophoresis (10% polyacrylamide, 8 M urea, 45 mM Tris-borate, 1 mM EDTA, pH 8.3), in which loaded quantities of ruthenium agent-treated DNA samples corresponded to approximately equal total radioactive counts visible on the gel. Crystallographic analysis of treated NCP NCP crystals were produced and stabilized in harvest buffer (37 mM MnCl 2 , 40 mM KCl, 20 mM K-cacodylate (pH 6.0), 24% 2-methyl-2,4-pentanediol and 2% trehalose) as previously described [37] . The 37-mM MnCl 2 buffer component was subsequently eliminated by gradual replacement with 10 mM MgSO 4 followed by thorough rinsing of crystals with the MgSO 4 -containing buffer to remove any residual MnCl 2 (ref. 8 ). The NCP–RAED-C crystal structure reported here stems from a 21-h incubation of NCP crystals with 1 mM RAED-C included in the buffer. Single-crystal X-ray diffraction data were recorded, with crystals mounted directly into the cryocooling N 2 gas stream set at −175 °C, at beam line X06DA of the Swiss Light Source (Paul Scherrer Institute, Villigen, Switzerland) using a Mar225 charge-coupled device (CCD) detector and an X-ray wavelength of 1.50 Å. Data were processed with MOSFLM [38] and SCALA from the CCP4 package [39] . The native NCP145 and NCP-TA2 models ( pdb codes 3REH and 3UTA) [4] , [25] were used for initial structure solution by molecular replacement. Structural refinement and model building were carried out with routines from the CCP4 suite [39] . Restraint parameters for the adducts were based on the small molecule crystal structure of RAED-C [16] . Data collection and structure refinement statistics are given in Table 4 . Graphic figures were prepared with PyMOL (DeLano Scientific LLC, San Carlos, CA, USA). Computational investigations We based our molecular dynamics (MD) simulations on the 2.5-Å resolution crystal structure of NCP (PDB code 3REH) [4] . We built four models using this structure as a reference, which differ in the site (DNA versus protein) in which the hydrolysed Ru drugs (RAED-C or RAPTA-C) were docked. Each model was immersed in a periodic box of ~130 × 97 × 133 Å 3 containing about 48,300 water molecules neutralized with Na + counterions. The box dimensions were chosen to achieve a minimum distance of 28 Å between two periodically replicated images of the system. The ff10 parameterization of the all-atom AMBER force field [40] , [41] , [42] , [43] was used to model protein residues, nucleic acids and counterions, whereas the TIP3P model [44] was employed for water molecules. Non-standard force field parameters for Ru drugs were taken from previous studies [45] . Electrostatic interactions were taken into account using the Particle Mesh Ewald algorithm [46] with a real-space cutoff of 12 Å. The same cutoff was employed for the treatment of the van der Waals interactions. An integration time step of 1 fs was used. Constant temperature (310 K) simulations were achieved by coupling the system to a Langevin thermostat. After initial minimization, systems were heated up to 310 K over 620 ps, while imposing positional restraints on the heavy atoms. Subsequently, restraints were slowly removed and 50 ns of unrestrained dynamics in the NVT ensemble were performed for each simulation to provide starting configurations for the following QM/MM runs. All the classical MD simulations were carried out using the NAMD package [47] . Four QM/MM MD simulations, one for each of the models equilibrated as mentioned above, were performed. Configurations in which the distance, d , between the Ru atom of RAPTA-C/RAED-C and the nucleophilic atom of the DNA site or histone site was ~8 Å were chosen to start the different QM/MM runs. The QM/MM implementation employed combines the use of the QM program QUICKSTEP [48] and the MM driver FIST, both part of the CP2 K package (freely available at the URL http://www.cp2k.berlios.de , released under GPL licence). In this code, the general QM/MM scheme is based on a real-space multigrid technique to compute the electrostatic coupling between both QM and MM regions [49] , [50] . In all the simulations, a quantum region consisting of the Ru compound and either the guanine base (truncation at the N9 atom) or the glutamate side chain (truncation at the C β atom) was treated at the density functional theory level. The remaining part of the system, including water molecules and counterions, was modelled at the classical level using the AMBER force field to take into account explicitly the steric and electrostatic effects of the macromolecular environment and solvent. The valence of the terminal QM atoms was saturated by the addition of capping hydrogen atoms, and a dual basis set, Gaussian and plane-wave formalism, was employed to compute the interaction energy within the QM subsystem. A molecularly optimized double-zeta valence basis set augmented with polarization functions (m-DZVP) was used [51] to describe the wave function, while an auxiliary plane-wave basis set expanded up to a density cutoff of 320 Ry was utilized to converge the electron density in conjunction with Goedecker–Teter–Hutter pseudopotentials [52] , [53] to describe the core electrons. Exchange and correlation energies were computed within the generalized gradient approximation by using the Perdew-Burke-Ernzerhof functional [54] . All the ab initio MD simulations were performed with Born–Oppenheimer MD in the canonical (NVT) ensemble and using an integration time step of 0.5 fs. The QM region of each of the QM/MM structures was initially relaxed by performing a geometry optimization while the MM part was kept frozen. Then the systems were thermalized and further equilibrated for about 2 ps by using a stochastic velocity rescaling thermostat [55] to maintain the temperature at 310 K. Snapshots extracted from these runs were used as starting configurations to estimate the free energy profiles corresponding to adduct formation on the DNA and histone sites for both Ru drugs. These free energy profiles were determined by integrating the constraint force acting along the distance d chosen as reaction coordinate [56] . For each value of the reaction coordinate, every system was run for 6–8 ps. Average forces were computed from data collected over the last 5 ps of those trajectories. Full QM calculations on model systems were carried out using the Gaussian09 suite of programmes [57] . Geometry optimizations were performed with the B3LYP density functional method [58] by using the relativistic effective core pseudopotential LANL2DZ for ruthenium and the 6-31+G* basis set for the remaining atoms [59] . To take into account condensed-phase effects, we used a united atom applied on radii optimized for Hartree-Fock [6-31G(d) level] polarizable continuum model with a relative permittivity of 78.3 to simulate bulk water effects [60] , [61] . Determination of cell growth inhibition parameters Human ovarian carcinoma cell lines, A2780 and crA2780, were purchased from the Health Protection Agency Culture Collections and maintained in culture as described above, with crA2780 cells additionally treated with 1 μM cisplatin for every 2–3 passages to maintain resistance. Cisplatin was purchased from Sigma-Aldrich, USA (P4394-250MG). To measure the cytotoxicity from exposure to different agents, cells were seeded in 96-well plates (5,000 cells per well) and grown for 24 h. Stock solutions of cisplatin, RAED-C, RAPTA-C were prepared in complete medium, subjected to serial dilutions and then added to the cells at various concentrations. Following a 72-h incubation, media were aspirated and 100 μl of 10% 3-(4,5-dimethylthiazol-2-yl)-2,5-diphenyltetrazolium bromide in RPMI complete medium (TOX1-1KT; MTT kit, Sigma-Aldrich, USA) was added to cells, which were incubated for 3 h at 37 °C. Subsequently, 100 μl of solubilization buffer was added to each well with vigorous pipetting to dissolve formazan. The resulting optical density was measured at 570 and 690 nm using a multi-well plate reader (Infinite M200 PRO, Magellan data analysis software; TECAN, Switzerland). The ratios of surviving cells were calculated by comparing with the untreated samples, and the IC 50 and IC 90 were derived based on three data sets (see Table 2 ). Cellular death and cell cycle analyses Cells were seeded into 35 mm-wells, incubated overnight and the following day cisplatin, RAED-C and RAPTA-C, were added into triplicate samples for 24 h incubations at concentrations corresponding to the IC 90 values. Subsequently, the media containing drugs was removed and fresh media was added. The cells were collected for analysis immediately (day 1) and subsequent to further 24 h (day 2) and 48 h (day 3) incubations in drug-free media. Extent of apoptosis/necrosis was assessed using an Annexin-V-FLUOS staining kit (11988549001; Roche Diagnostics, Germany). Floating cells as well as attached cells were collected, washed in PBS and stained with Annexin V and propidium iodide. Cells were then incubated for 15 min in the dark and analysed on an LSR II flow cytometer (BD FACSDiva software, BD Biosciences). For the cell cycle analysis, cells were rinsed in PBS, trypsinized, pelleted and washed before they were added in a drop-wise manner into 70% ethanol. After overnight incubation, cells were washed in PBS and incubated with 4',6-diamidino-2-phenylindole dihydrochloride (3 μM, Life Technologies) for 15 min in the dark before analysing on an LSR II flow cytometer (BD FACSDiva software, BD Biosciences). Analysis of cellular data was based on three independent replicates of each experiment. Graphic plots were generated with Excel (Microsoft Corporation). Mahalanobis multivariate analysis was carried out using Xlstat (version 2013.1.01; Addinsoft Corporation). How to cite this article: Adhireksan, Z. et al. Ligand substitutions between ruthenium–cymene compounds can control protein versus DNA targeting and anticancer activity. Nat. Commun. 5:3462 doi: 10.1038/ncomms4462 (2014). Accession codes: Atomic coordinates and structure factors have been deposited in the Protein Data Bank under accession code 4KGC .